Navigable networks as Nash equilibria of navigation games Common sense suggests that networks are not random mazes of purposeless connections, but that these connections are organized so that networks can perform their functions well. One function common to many networks is targeted transport or navigation. Here, using game theory, we show that minimalistic networks designed to maximize the navigation efficiency at minimal cost share basic structural properties with real networks. These idealistic networks are Nash equilibria of a network construction game whose purpose is to find an optimal trade-off between the network cost and navigability. We show that these skeletons are present in the Internet, metabolic, English word, US airport, Hungarian road networks, and in a structural network of the human brain. The knowledge of these skeletons allows one to identify the minimal number of edges, by altering which one can efficiently improve or paralyse navigation in the network. Networks are efficient conduits of information and other media. News, ideas, opinions, rumours and diseases spread through social networks fast, sometimes becoming viral for reasons that are often difficult to predict [1] , [2] , [3] , [4] , [5] , [6] , [7] , [8] , [9] , [10] , [11] , [12] . Many biological networks are also paradigmatic examples of information routing, ranging from information processing and transmission in the brain, to signalling in gene regulatory networks, metabolic networks or protein interactions [13] , [14] , [15] , [16] . Perhaps the most basic example is the Internet whose primary function is to route information between computers. If one is to list some common functions of different networks, then information routing will likely be close to the top. It is thus not surprising that many networks were found navigable, meaning that nodes can efficiently route information through the network even though its global structure is not known to any individual node [17] , [18] , [19] , [20] , [21] , [22] , [23] , [24] , [25] , [26] , [27] , [28] . These findings do not necessarily mean that real networks evolve to become navigable. Navigability can be a by-product of some other evolutionary incentives because different networks have many other different functions as well. In other words, it remains unclear whether ideal networks whose only purpose is to be maximally navigable at minimal costs have anything in common with real networks. Even if they do, then how close are real networks to these ideal maximally navigable configurations? If they are close but not exactly there, or if their navigability suddenly deteriorates, possibly signifying an onset of a disease [29] , then what can we do to cure the network and boost its navigability? Here we show that the ideal maximally navigable networks do share some basic structural properties with the Internet, E.coli metabolic network, English word network, US airport network, the Hungarian road network and a structural network of the human brain. Yet these ideal networks are not generative models of the real networks, where by generative models we mean function-agnostic models that simply try to reproduce some structural properties of real networks. Instead these ideal networks identify minimal sets of edges that are most critical for navigation in the real network. In other words, they are navigation skeletons or subgraphs of real networks. We find that the considered real networks contain high percentages, exceeding 90% in certain cases, of edges from their navigation skeletons, while the probability of such containment in randomized null models is exponentially small. The knowledge of these skeletons allows us to quantify exactly what connections the considered real networks lack to be maximally navigable, and which of their connections are not exactly necessary for that. To define and construct these maximally navigable network skeletons we employ game theory. Game theory is a standard tool to study the behaviour of a population with given incentives. The population members are called players, and their possible actions are strategies, while cost functions or payoffs express players’ incentives. The purpose of a player is to minimize her costs (or maximize her payoffs) by adjusting her strategy. A Nash equilibrium is a game state such that no player can further reduce her costs by altering her strategy unilaterally. Such equilibrium states are local optima where the game can eventually settle after some transient dynamics. The global optimum is an optimum where the total cost of all players is minimized. Since the inception of game theory a broad palette of games has been introduced, modelling diverse properties of real-life situations [30] , Fig. 1 . Here we use game theory to find the structure of networks that are Nash equilibria of a network construction game [30] , [31] , [32] , [33] , [34] , [35] , [36] with navigability incentives. The concept of Nash equilibrium captures the idea of self-organization, that is, of the emergence of structures from the local interaction of rational but selfish players, in contrast to global optimization used in centralized planning of globally optimal navigable structures [37] . In our network navigation game (NNG), players are network nodes whose optimal strategy is to set up a minimal number of edges to other nodes ensuring maximum navigability. That is, the cost function reflects trade-offs between the number of created edges and navigability. If each node connects to each other node, then this construction is maximally navigable but maximally expensive too. If no edges are set up, then the cost is zero, but so is navigability. There is a sweet spot of the least expensive but still 100% navigable network, defined as the network in which all pairs of nodes can successfully communicate using geometric routing [38] . The goal of our game is to find this sweet spot. 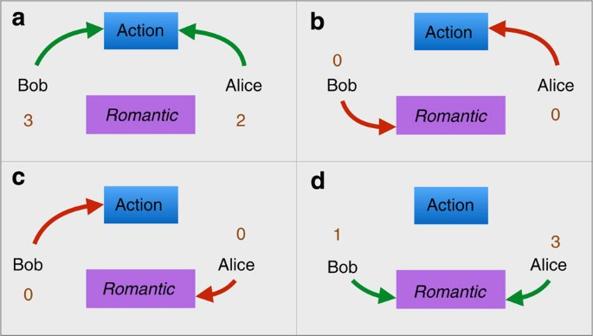Figure 1: Illustration of game theory. Alice and Bob are happy only if they go out to the movies together, but the level of their happiness depends on what movie they watch. The basic notions of a game: Players: Alice and Bob; strategies: go to see an action or a romantic movie; payoffs: the level of happiness 0,1,2,3; Nash equilibria: situations in which the players cannot be happier by unilaterally modifying their strategies. Among all the possible states (a–d) in the figure, states (a) and (d) are equilibria when Alice and Bob go together to watch a movie. State (a) is the global optimum since the total happiness 3+2=5 is maximized. Figure 1: Illustration of game theory. Alice and Bob are happy only if they go out to the movies together, but the level of their happiness depends on what movie they watch. The basic notions of a game: Players: Alice and Bob; strategies: go to see an action or a romantic movie; payoffs: the level of happiness 0,1,2,3; Nash equilibria: situations in which the players cannot be happier by unilaterally modifying their strategies. Among all the possible states ( a – d ) in the figure, states ( a ) and ( d ) are equilibria when Alice and Bob go together to watch a movie. State ( a ) is the global optimum since the total happiness 3+2=5 is maximized. Full size image Geometrical considerations The network construction game that we employ is very general and applies to any set of points in any geometry. The latent geometry of numerous real networks is not Euclidean but hyperbolic as shown in ref. 39 . Specifically, the model in ref. 39 extends the preferential attachment mechanism of network growth by observing that in many real networks the probability of establishing a connection depends not only on popularity of nodes, that is, their degrees, but also on similarity between nodes. Similarity is modelled in ref. 39 as a distance between nodes on the simplest compact space, the circle. The connection probability thus depends both on node degrees (popularity) and on the distance between nodes on the circle (similarity). The node degrees are then mapped to radial coordinates of nodes, thus moving nodes from the circle to its interior, the disk. One can then show that the resulting connection probability depends only on the hyperbolic (versus Euclidean) distance between nodes on the disk, and that the resulting graphs are random geometric graphs [40] growing over the hyperbolic plane. As shown in earlier work [41] , these graphs are maximally random, that is, maximum-entropy graphs that have power-law degree distributions and strong clustering. In other words, power-law degree distributions, coupled with strong clustering, are manifestations of latent hyperbolic geometry in networks. If this geometry is not hyperbolic but Euclidean, then the resulting random geometric graphs still have strong clustering, but their degree distributions are Poisson distributions that do not have any fat tails [40] . The model in ref. 39 has been validated against long histories of growth of several real networks, predicting their growth dynamics with a remarkable precision. It is then not surprising that as a consequence the same model also reproduces a long list of structural properties of these networks [39] . Random geometric graphs [40] are defined as sets of points sprinkled uniformly at random over a (chunk of) geometric space. Every pair of points is then connected if the distance between the points in the space is below a certain threshold. Given that the latent space of real scale-free networks is hyperbolic, our starting point is the first part (uniform sprinkling) of the random geometric graph definition. That is, we first randomly sprinkle a set of points over a hyperbolic disk. We then do not proceed to the second part of the random geometric graph definition. Instead, given only the coordinates of sprinkled nodes, we identify the sets of edges, ideal for navigation, that correspond to the Nash equilibria of our NNGs. We then analyse the structural properties of the resulting ideal-navigation networks, and find that, surprisingly, they also have power-law degree distributions and strong clustering. This result invites us to investigate whether these navigation-critical edges exist in real networks. To check that, we have to know the hyperbolic coordinates of nodes in these real networks in the first place. We infer these coordinates in the considered collection of real networks using the deterministic HyperMap algorithm (Methods). Given only these inferred coordinates, we then construct the ideal-navigation Nash equilibria defined by these coordinates, and compare, edge by edge, the resulting Nash equilibrium networks against the real networks. We find that the real networks contain large percentages of edges from their Nash equilibria. This methodology thus allows us to identify the navigation skeleton of a given real network. We finally check directly that edges in these skeletons are indeed most critical for navigation by showing that their alterations affect markedly network navigability. Game definition We start with a set of players u =1,2,…, N , that is, N nodes, scattered randomly over a hyperbolic disk of radius R . The densities of players’ polar coordinates ( r , φ ), r ∈ [0, R ], φ ∈ [0, 2 π ], are [41] where α >1/2 is a parameter controlling the heterogeneity of the layout. If α =1, the players are distributed uniformly over the hyperbolic disk because the area element at coordinates ( r , φ ) is dA =sinh( r ) dr dφ . The desired player scattering is achieved in simulations by placing players u at polar coordinates r u =(1/ α ) acosh {1+[cosh( αR )−1] U } and φ u =2 πU where U for each u is a random number drawn from the uniform distribution on [0, 1]. The hyperbolic distance between any two players u and v is In greedy geometric routing, player u routes information to some remote player v by forwarding the information to its connected neighbour u ′ closest to v in the plane according to the distance above. If u has no neighbour u ′ closer to v than u self, then navigation fails, and we say that u cannot navigate to v . The percentage of pairs of players u , v such that u can successfully navigate to v is called the success ratio. If this percentage is 100%, we say that the network is maximally (100%) navigable. The strategy space of player u is all possible combinations of edges that u can establish to other players. One extremal strategy is to establish no edges. The other extreme is to connect to everyone. The total number of possibilities for u is 2 N −1 . Any combination of strategies that all players select is a network on N nodes. The objective of each player u is to set up a minimal number of edges to other players such that u can still navigate to any other player in the network. Formally, the cost function of player u that it minimizes is c u = k u + n u , where k u is the number of edges that u establishes, and n u is either zero if u can navigate to everyone, or infinity otherwise. A more formal description of the strategies and payoffs can be found in Supplementary Note 1 . Nash equilibria of the game Given any player u , we call player v 's coverage area the set of all points closer to v than to u , Fig. 2 . Trivially v covers itself, since it is closer to itself ( d ( v , v )=0) than to u . Therefore if u connects to all other players, then u trivially covers them all. The optimal strategy for u minimizing u 's costs is thus to connect to a minimal number of players such that the union of their coverage areas contains all the other players. Indeed, if u does that, and if all other players do the same, then the resulting network is 100% navigable at minimal number of edges. The network is fully navigable because if u wants to navigate to any remote player w , then by construction there exists u 's neighbour v that contains w in its coverage area, and u can use v as the next hop towards w . If v is not directly connected to w , then there exists v 's neighbour v ′ that contains w in its coverage area, so that v can route to v ′, and so on until the information reaches destination w lying within the intersection of all the coverage areas along the path, Fig. 2 . The problem of finding the optimal set of edges for u thus reduces to the minimum set cover problem [42] . A formal description of the equilibrium network and a detailed example (for simplicity in the Euclidean plane) can be found in Supplementary Note 2 and Supplementary Fig. 1 . 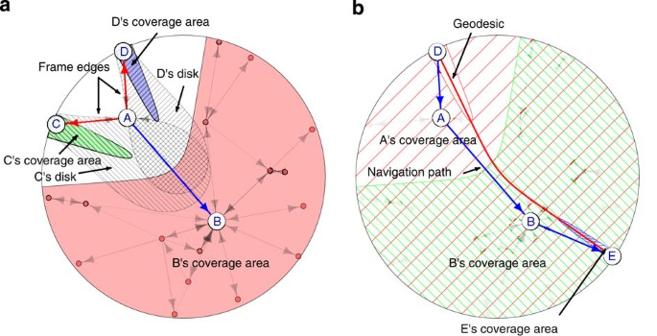Figure 2: Illustration of the network navigation game (NNG). Panel (a) shows the optimal set of connections (optimal strategy) of node A in a small simulated network. All nodes are distributed uniformly at random over the hyperbolic disk, and A’s optimal strategy is to connect to the smallest number of nodes ensuring maximum (100%) navigability. These nodes are B, C and D because it is the smallest set of nodes whose coverage areas, shown by the coloured shapes, contain all other nodes in the network. B’s coverage area for A (red) is defined as a set of points hyperbolically closer to B than to A; therefore, if A is to navigate to any point in this area, A can select B as the next hop, and the message will eventually reach its destination, as the second panel illustrates. Link AC (and AD) in panel (a) is also a frame link, because A is the closest node to C, as illustrated by the hyperbolic disk of radius |AC| centred at C (the line-filled shape), which does not contain any nodes other than C and A. Therefore, to navigate to C, A has no choice other than to connect directly to C. Panel (b) shows the sequence of shrinking coverage areas along the navigation path (blue arrows) from D to E. The red curve is the geodesic between D and E in the hyperbolic plane. The coverage areas are shown by the shapes filled with lines of increasing density. The largest is A’s coverage for D. The next one is B’s coverage for A. The smallest is E’s coverage for B. Figure 2: Illustration of the network navigation game (NNG). Panel ( a ) shows the optimal set of connections (optimal strategy) of node A in a small simulated network. All nodes are distributed uniformly at random over the hyperbolic disk, and A’s optimal strategy is to connect to the smallest number of nodes ensuring maximum (100%) navigability. These nodes are B, C and D because it is the smallest set of nodes whose coverage areas, shown by the coloured shapes, contain all other nodes in the network. B’s coverage area for A (red) is defined as a set of points hyperbolically closer to B than to A; therefore, if A is to navigate to any point in this area, A can select B as the next hop, and the message will eventually reach its destination, as the second panel illustrates. Link AC (and AD) in panel ( a ) is also a frame link, because A is the closest node to C, as illustrated by the hyperbolic disk of radius | AC | centred at C (the line-filled shape), which does not contain any nodes other than C and A. Therefore, to navigate to C, A has no choice other than to connect directly to C. Panel ( b ) shows the sequence of shrinking coverage areas along the navigation path (blue arrows) from D to E. The red curve is the geodesic between D and E in the hyperbolic plane. The coverage areas are shown by the shapes filled with lines of increasing density. The largest is A’s coverage for D. The next one is B’s coverage for A. The smallest is E’s coverage for B. Full size image The Nash equilibrium of this game is not necessarily unique. There can exist different networks minimizing the cost defined above. As specified in Supplementary Note 2 , in what follows, among all the NNG equilibria, we always select the unique one that minimizes the sum of distances span by its edges, thus making the NNG Nash equilibrium network construction deterministic. However, there also exist certain edges, which we call frame edges, necessarily present in any Nash equilibrium. Edge u → v is a frame edge if u is the closest player to v . In this case u cannot navigate to v through any other players since there is no one closer to v than u self, so that u must connect directly to v to reach it, Fig. 2 . If at least one of such edges is absent, the network is not fully navigable. The exact definition of the ‘frame topology’ consisting the frame edges can be found in Supplementary Note 3 and Supplementary Fig. 2 . In any Nash equilibrium of this game, each player computes its optimal strategy independently of others. In game theory such equilibria are called dominant strategy equilibria. Moreover, the equilibrium is also a social optimum since one cannot create a fully navigable network using less edges. Structural properties of Nash-equilibrium networks Using the trigonometry of overlapping hyperbolic disks, we show in Supplementary Note 4 and Supplementary Figs 2–6 that, if the node density is uniform ( α =1), then the probability p ( d ) that two players u and v located at distance d ≡ d ( u , v ) are connected in a Nash equilibrium network lies between exp(−8 δe d /2 ) and exp(−2 δe d /2 ), where δ is the average density of players on the disk, that is δ = N / A , where A is the disk area. The expected degree of player u at polar coordinates ( r u , 0)—we can assume that u 's angular coordinate is φ u =0 without loss of generality—is then , where ρ ( r v ) and ρ ( φ v ) are the player densities from Equation 1. We can evaluate this integral to find that the expected number of connections of a player at radial coordinate r is bounded by (analytically shown in Supplementary Note 5 and Supplementary Fig. 7 ) where r ≡ r u . It then follows that the average degree of players in the network, given by , lies between 1 and 4, We also see from Equation 4 that the degree of players decays exponentially as the function of their radial position, , while their density exponentially increases, ρ ( r ) ∼ e r , Equation 1. The combination of these two exponentials yields the power-law degree distribution (see Supplementary Note 6 and Supplementary Fig. 8 for the detailed derivation) in the network [43] , [44] We also show analytically in Supplementary Note 7–8 , Supplementary Fig. 9 and Supplementary Table 1 that the average clustering of players of degree k decays with k as 1/ k , while the average clustering in the network is around 0.45, also confirmed in simulations. Clustering does not depend on network size or average degree, meaning that clustering is a positive constant even in the large graph size limit. Remarkably, neither degree distribution nor clustering depends on the player density δ . For non-uniform node density α ≠1, we can analytically obtain only the lower bound for , which is still proportional , that is, independent of α if α >1/2, Supplementary Note 9 . This lower bound suggests that the degree distribution is a power law P ( k ) ∼ k − γ with exponent γ =2 α +1, which we confirm in simulations in Supplementary Note 9 and Supplementary Fig. 10 . 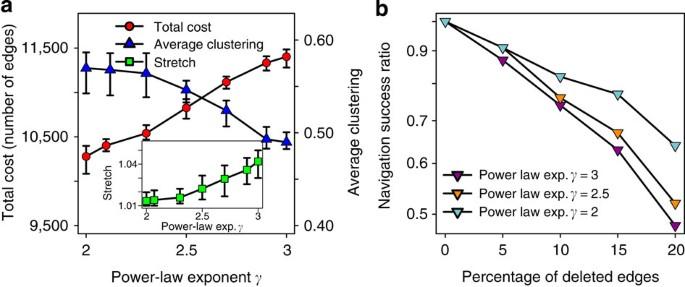Figure 3: Topological properties of NNG equilibrium networks as a function of the power-law exponent. Panel (a) shows the total cost (number of edges), average clusteringand stretch in NNG-simulated networks as functions of γ. Stretch (shown in the inset) is the average factor showing by how much longer the greedy navigation paths are, compared with the shortest paths in the network. Stretch equal to 1 means that all navigation paths are shortest possible. The plotted points are mean values while the error bars show minimum and maximum values obtained for the NNG over 10 random sprinkling of nodes for a given value ofγ. Panel (b) shows the success ratio as a function of the percentage of edges randomly deleted from the network. The smaller theγ, the more robust the navigability with respect to this network damage. Figure 3 shows that the closer the γ to 2, the stronger the clustering, the cheaper the network and the more efficient and robust the navigability. The value of γ =2 thus appears as the ‘best choice’ for a network—the network is maximally navigable at the lowest cost. These results complement existing works [23] , [45] showing that γ =2 yields most navigable networks, by adding that this γ also provides a minimum cost equilibrium topology as well, explaining the emergence of these networks from the interaction of selfish players. Figure 3: Topological properties of NNG equilibrium networks as a function of the power-law exponent. Panel ( a ) shows the total cost (number of edges), average clustering and stretch in NNG-simulated networks as functions of γ. Stretch (shown in the inset) is the average factor showing by how much longer the greedy navigation paths are, compared with the shortest paths in the network. Stretch equal to 1 means that all navigation paths are shortest possible. The plotted points are mean values while the error bars show minimum and maximum values obtained for the NNG over 10 random sprinkling of nodes for a given value of γ . Panel ( b ) shows the success ratio as a function of the percentage of edges randomly deleted from the network. The smaller the γ , the more robust the navigability with respect to this network damage. 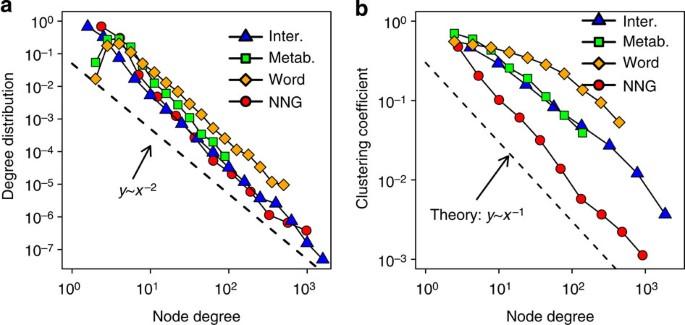Figure 4: NNG equilibrium networks share basic structural properties with real networks. The real networks considered are the Internet, metabolic reactions, and the English word network, see Methods. Panels (a,b) show the degree distribution and the average clustering coefficient of nodes of a given degree in the real and NNG networks. The dashed black lines are the power laws with exponents −2 and −1. The power law decay of the clustering coefficient for the NNG is shown analytically inSupplementary Note 7. The clustering coefficient of a node of degreekis the number of triangular subgraphs containing the node, divided by the maximum possible such number, which isk(k−1)/2. In the NNG network, the disk radius isR=21.2 andα=0.5. There are no other parameters. Full size image Figure 4 and Table 1 confirm our analytic results and shows that some basic structural properties of NNG-simulated networks are similar to some real networks. Our results also suggest that the incentive for navigability alone may be sufficient to explain the properties of complex networks to a certain degree. Yet we cannot really make this claim based only on such large-scale statistical similarities. A more detailed link-by-link comparison between real and corresponding NNG networks is needed to understand how well the NNG reflects reality. Figure 4: NNG equilibrium networks share basic structural properties with real networks. The real networks considered are the Internet, metabolic reactions, and the English word network, see Methods. Panels ( a , b ) show the degree distribution and the average clustering coefficient of nodes of a given degree in the real and NNG networks. The dashed black lines are the power laws with exponents −2 and −1. The power law decay of the clustering coefficient for the NNG is shown analytically in Supplementary Note 7 . The clustering coefficient of a node of degree k is the number of triangular subgraphs containing the node, divided by the maximum possible such number, which is k ( k −1)/2. In the NNG network, the disk radius is R =21.2 and α =0.5. There are no other parameters. Full size image Table 1 Comparison of basic structural properties of real and NNG networks. 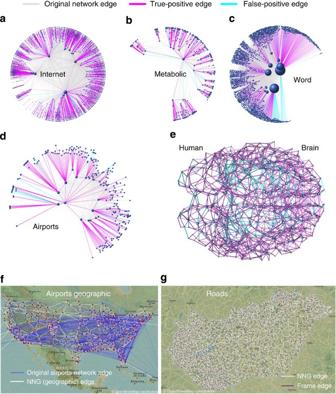Figure 5: Network navigation game predicts well links in real networks. Panels (a–c) visualize the Internet, metabolic and word networks mapped to the hyperbolic plane as described in the Methods section. The hyperbolic coordinates of nodes are then supplied to the minimum set cover algorithm that finds a Nash equilibrium of the NNG for each network. Panels (d,e) do the same for the US airport network and for the human brain, except that in the brain the physical coordinates of nodes are used. The grey edges are present in the real networks but not in the NNG networks. These edges may exist in real networks for different purposes other than navigation, so that the NNG can say nothing about them. The false-positive turquoise edges are present in the NNG networks but not in the real networks. The true-positive magenta edges are present in both networks. Panels (f,g) show the NNG equilibrium network based on the physical (geographic, versus hyperbolic) coordinates of US airports, and the NNG network for the Hungarian road network. The NNG networks have the same sets of nodes as the corresponding real networks, but the sets of edges are different. For visualization purposes the grey edges are suppressed in the human brain and Hungarian road networks. The detailed statistics of edges are inTable 2. The cartography in the background of panels (f,g) have been generated with OpenStreetMap, © OpenStreetMap contributors (seewww.openstreetmap.org/copyrightfor details). Full size table Network navigation game versus real networks Figure 5 and Table 2 show the results of this analysis applied to these and other real networks. We cannot expect real networks to be identical to NNG networks because the latter are minimum-cost maximum-navigation idealizations, while each individual real network performs many other functions different from navigation. In particular, since real networks must be error-tolerant and robust with respect to different types of network damage, we expect the number of edges in real networks to be noticeably larger than that in their minimalistic NNG counterparts—something we indeed observe in Table 2 . Yet if navigation efficiency does matter for real networks, then we should expect a majority of edges present in these NNG idealizations to be also present in the corresponding real networks. Table 2 confirms these expectations as well. The NNG precision in predicting links in real networks, defined as the ratio of NNG true positive links to the total number of NNG links, exceeds 80% for most networks, while the precision in predicting frame links, crucial for navigation, exceeds 90% for some networks. In Supplementary Note 10 we juxtapose these numbers against the corresponding numbers in randomized null models, where they are exponentially small, upper bounded by 0.1%. We also note that, as the real networks have many more links than NNG networks, their navigability may not suffer much from missing a small percentage of NNG links, as confirmed by the success ratio results in the same figure. Figure 5: Network navigation game predicts well links in real networks. Panels ( a – c ) visualize the Internet, metabolic and word networks mapped to the hyperbolic plane as described in the Methods section. The hyperbolic coordinates of nodes are then supplied to the minimum set cover algorithm that finds a Nash equilibrium of the NNG for each network. Panels ( d , e ) do the same for the US airport network and for the human brain, except that in the brain the physical coordinates of nodes are used. The grey edges are present in the real networks but not in the NNG networks. These edges may exist in real networks for different purposes other than navigation, so that the NNG can say nothing about them. The false-positive turquoise edges are present in the NNG networks but not in the real networks. The true-positive magenta edges are present in both networks. Panels ( f , g ) show the NNG equilibrium network based on the physical (geographic, versus hyperbolic) coordinates of US airports, and the NNG network for the Hungarian road network. The NNG networks have the same sets of nodes as the corresponding real networks, but the sets of edges are different. For visualization purposes the grey edges are suppressed in the human brain and Hungarian road networks. The detailed statistics of edges are in Table 2 . The cartography in the background of panels ( f , g ) have been generated with OpenStreetMap, © OpenStreetMap contributors (see www.openstreetmap.org/copyright for details). Full size image Table 2 The table quantifies the relevant edge statistics in Fig. 5 , showing the total number of edges in the real networks | R |, and in their NNG equilibrium networks | M |, the number of true positive (magenta edges in Fig. 5 ) | T |=| M ∩ R |, the number of false positive (turquoise edges in Fig. 5 ) | F |=| M \ R |, and the true positive rate, or precision, defined as | T |/| M |. Full size table Of particular interest to us here are networks that are explicitly embedded in the physical space. In these cases we may not need to embed the network, but use instead the physical coordinates of its nodes to construct the NNG equilibria. We consider three examples: the Hungarian road network, the airport network of the United States and a structural network of the human brain. In the first network the nodes are the cities, towns and villages of Hungary, while in the second network the nodes are US airports. Two nodes are linked if they are connected by a direct road or flight. In the brain network the nodes are small regions of average size 1.5 cm 2 covering entirely both hemispheres of the cerebral cortex, and two regions are connected if a structural connection between them is detected in diffusion spectrum imaging. We expect the NNG to be particularly accurate in predicting links in these networks using the physical—instead of hyperbolic—coordinates of nodes. We note that these physical coordinates are Euclidean in all the three cases. The embedding space is two-dimensional Euclidean and spherical space in the road and airport cases, and it is three-dimensional Euclidean space in the brain case. Our method to construct an NNG equilibrium applies without change to any set of points in any geometric space, and the analytic results on the structure of NNG equilibrium networks in Euclidean spaces are in Supplementary Note 11 and Supplementary Fig. 11 . We apply our method to find the NNG equilibrium networks using the physical coordinates of nodes in these three real networks, and then compare them with their NNG equilibria also in Fig. 5 and Table 2 . We observe that in the brain and road networks the NNG link prediction accuracy is particularly high, reaching 89% for all the links and 94–95% for the frame links. For the brain this result implies that the spatial organization of the brain is nearly optimal for information transfer, in agreement with previous results [46] , [47] , [48] , [49] . In the Hungarian road network, nearly all frame links, crucial for efficient navigation using geography, are present. Practically this means that Hungarians have luxury to go on a road trip without a map since all the major roads required by geographic navigation are there, albeit the condition of some of those roads is not as luxurious. To put it simply, there are roads where people with a compass may think they should be. For the US airport network, however, the geographic results are poor. These poor results may be unexpected at first, but they have a simple explanation in that the geometry of the airport network is not really Euclidean, as the geometry of the nearly planar road network, but hyperbolic. Indeed, efficient paths in the airport network optimize not so much the geographic distance travelled, but the number of connecting flights. As a consequence, most paths go via hubs. As opposed to the road network, where the number of roads meeting at an intersection does not vary that much from one intersection to another, the presence of hubs in the airport network makes the network heterogeneous, that is, node degrees vary widely. This heterogeneity effectively creates an additional dimension (the ‘popularity’ dimension in ref. 39 ). That is, in addition to their geographic location, airports also have another important characteristic—the size or degree. This extra dimension makes the network hyperbolic [41] . The NNG results for the hyperbolic map of the airport network in Fig. 5 are as good as for the other networks. How to cure or injure a network efficiently The knowledge of the NNG equilibrium of a given real network makes it possible to efficiently identify links that are most critical for navigation in the network. As NNG equilibrium networks are maximally navigable networks composed of the smallest number of links, we expect that if we alter a real network by either adding or removing a relatively small number of links belonging to the NNG equilibrium of the network, then such network modifications may significantly affect network navigability. 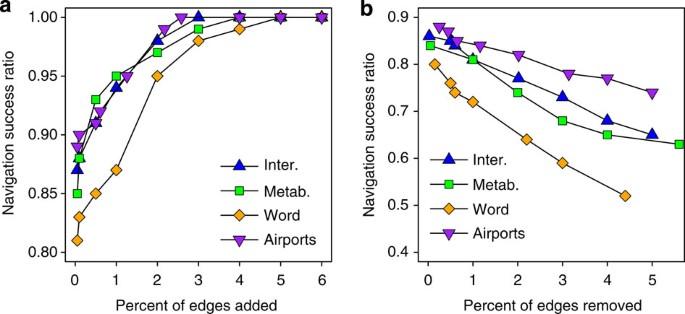Figure 6: NNG equilibria of real networks helps to improve or degrade their navigability. The edges from the NNG equilibria of the considered real networks are first sorted in the decreasing order of betweenness centrality, and then either added to the real network if not already there (panel (a)), or removed from the network if present (panel (b)). Thex-axis shows the percentage of added or removed edges compared with the number of edges in the original real network. Navigation success ratio is computed as the number of node pairs between which geometric routing is successful divided by the number of all node pairs. Figure 6 supports these expectations. In the figure, we take the considered real networks, and add to them certain numbers of links that are present in the NNG equilibria of the real networks, but not present in the networks themselves. About 1–2% of added edges, compared with the original numbers of edges in the networks, increase network navigability significantly, while the addition of 2–5% of edges makes all the networks 100% navigable. Similarly, the targeted removal of a small portion (1–5%) of edges belonging both to the NNG equilibria of the networks, and to the network themselves, degrades network navigability by 10–30%. Figure 6: NNG equilibria of real networks helps to improve or degrade their navigability. The edges from the NNG equilibria of the considered real networks are first sorted in the decreasing order of betweenness centrality, and then either added to the real network if not already there (panel ( a )), or removed from the network if present (panel ( b )). The x -axis shows the percentage of added or removed edges compared with the number of edges in the original real network. Navigation success ratio is computed as the number of node pairs between which geometric routing is successful divided by the number of all node pairs. Full size image We emphasize that the considered Nash equilibrium networks are minimalistic idealizations, concerned only with maximizing the efficiency of the navigation function at minimal cost (number of links). Reality differs from this ideal in many ways. First, real networks must be robust with respect to noise and random failures. This robustness requirement explains why the considered real networks have strictly more links than their Nash equilibria. Maximum navigability can obviously be achieved not only at the minimal cost, but also at a higher cost. Second, transport processes in real networks are also noisy, and can follow not only steepest descent path (greedy navigation), but also any downstream paths, still achieving 100% reachability. Yet the noisier the transport process, the less likely it stays to the shortest path, leading to higher stretch and longer travel times, thus degrading navigation efficiency in terms of these parameters. Third, navigability does not always have to be maximized as many specific networks perform many specific functions other than navigation. Our game-theoretic approach can be extended to accommodate some of these functions, such as error tolerance or policy compliance [50] , but not all possible functions of different real networks can be formalized within this game-theoretic framework. Some networks are centrally designed to optimize a particular function globally [37] . Game theory is not needed to formalize such global optimization strategies. It is more suited for self-organized networks, in which each node behaves selfishly according to its own incentive, independent of other nodes. In other words, Nash equilibrium networks are structural manifestations of local incentives of nodes for efficient transport or communication, in contrast with existing generative or optimization models of complex networks [51] , [52] . Finally, all real networks are dynamic and growing, while Nash equilibria correspond to static network configurations. However, it has been recently shown [53] that in case of random geometric graphs—to which the considered Nash equilibrium networks effectively belong according to the results in Supplementary Note 12 —one can map an equilibrium network model to an identical growing one. Notwithstanding these limitations we have shown that ideal networks designed to be maximally navigable at minimal cost share basic structural properties with real networks. Compared with existing works on navigation-optimal distributions of shortcut edges in Euclidean grids [19] , [54] , [55] , [56] , which do not yield realistic network topologies, this result is quite unexpected because there is absolutely nothing in the definition of these ideal networks that would enforce or even welcome a formation of any particular network structure. The networks are defined purely in terms of navigation optimality. The surprising finding that the structure of these ideal networks is similar to the structure of real networks should not be misinterpreted as if these idealizations are generative models for real navigable networks. Instead the former are skeletons or subgraphs of the latter. Since these skeletons consist of the minimum number edges required for 100% navigability, there is not even a parameter to control the most basic structural network property—the average degree, which is always controllable in generative models. On the contrary, as follows from Equation 5, the average degree in these skeletons is uncontrollable and lies between 1 and 4. We find that, if network geometry is hyperbolic, then our navigation skeletons have power-law degree distributions and strong clustering. The values of power-law exponent γ close to 2, observed in many real networks [57] , [58] , appear as the best possible choice. In this case not only reachability is 100%, but also the network cost and stretch are minimized and navigability robustness is maximized, compared with other values of γ in Fig. 3 . These results apply to sets of points in hyperbolic space, but the navigation skeleton construction itself is by no means limited to these hyperbolic settings. It is very general, and applies to any set of points in any geometric space, as illustrated by the brain and road networks where we have used the Euclidean 2 d and 3 d physical coordinates of nodes to construct the navigation skeleton of the network. Our finding that the brain contains almost fully its navigation skeleton appears as a mathematically clear and conclusive evidence that the spatial organization of the brain is nearly optimal for communication and information transfer, corroborating existing work on the subject [46] , [47] , [48] , [49] . We note that the connection between the structure and function of networks is often studied in the logically reverse direction: structure→function. That is, first some data about the structure of real networks is obtained, and then questions concerning how optimal this structure is with respect to a given network function are investigated. This logic does provide some evidence that the network might have evolved optimizing this function, but this evidence is quite indirect and unreliable compared with the direct demonstration that functionally optimal networks have the structure observed in reality: function→structure. The common sense suggests that this causal direction must reflect reality more adequately as networks, either designed or naturally evolving, do not have a completely random structure but the structure (effectively) optimizing some functions. Yet studying networks in this direction is much more challenging primarily because of difficulties in formalizing the constraints that a given function imposes and deriving the resulting optimal network structure. Here, with the help of game theory, we have done so for the navigation function that many real networks (implicitly) perform. As one would logically expect, the function→structure approach provides a deeper insight into specific details of network’s structural organization that are critical for its functional efficiency. We have confirmed this expectation by demonstrating that our approach can identify links in real networks that are most critical for navigation. A targeted attack on these critical links degrades navigability rapidly, while if a real network is not 100% navigable, our approach finds the minimal number of not-yet-existing links whose addition to the network boosts up its navigability to 100%. Therefore, our approach can be used to identify real network links that should be protected most in a critical network infrastructure. In contrast, this approach can also help network designers to prioritize possible link placement options, that is, pairs of not directly connected nodes, that, if connected, would maximize navigability improvement. Finally, all the real networks considered here are expected to be navigable. Indeed, the primary functions of the Internet, brain, metabolic or airport and road networks are to transport information, energy or people. Semantic and syntactic navigability of word networks is an established fact in cognitive science [59] , [60] , [61] . However, one cannot expect all real networks to be highly navigable as navigation is not an important function of every network in the world. In Supplementary Note 13 and Supplementary Table 2 we consider one example, a technosocial web of trust, in which nodes are public keys of users of a distributed cryptosystem, linked by users’ certifications of key-user bindings. There is no reason why this network should be navigable. In agreement with this observation, we then find that this network does not contain a large percentage of edges from its NNG equilibrium, suggesting that the introduced methodology can be also used as a litmus test to investigate whether navigation is an important function of a given real network, and if so, then to what degree. The real network data The Internet data set representing the global internet structure at the autonomous system (AS) level is from ref. 62 . The metabolic network is the post-processed network of metabolic reactions in E. coli from ref. 39 , Snapshot S 1 there. The post-processing details can be found in ref. 39 . The word network is the largest connected component of the network of adjacent words in Charles Darwin’s ‘The Origin of Species’ from ref. 63 . The airport network was downloaded from the Bureau of Transportation Statistics http://transtats.bts.gov/ on 5 November 2011. The structural human brain network and physical coordinates of nodes (regions of interest (ROIs)) in it are the diffusion spectrum imaging (DSI) data from ref. 64 . The hyperbolic maps of real networks The hyperbolic coordinates of ASes and metabolites are from refs 39 , 62 . The hyperbolic coordinates of words and airports are inferred using the HyperMap algorithm [65] . This algorithm is deterministic and is based on the growing network model in ref. 39 used to show that the latent geometry of scale-free strongly clustered real networks is hyperbolic. Given an adjacency matrix of a real network, the algorithm infers the hyperbolic coordinates of its nodes by replaying its growth as the model in ref. 39 prescribes. Specifically, the nodes are first sorted in the order of decreasing degrees, and then, starting with the highest-degree node, nodes and their edges are added, one node at a time, to a growing network. The probability, or the likelihood, with which model [39] generates this growing network, depends on the node coordinates. The coordinate of each added node is set by the HyperMap algorithm to the coordinate corresponding to the global maximum of this probability. The Nash equilibrium networks of NNGs The hyperbolic or physical, in the airport and brain cases, coordinates are then supplied to the GNU Linear Programming Kit (GLPK) http://www.gnu.org/software/glpk/ used to find a solution to the corresponding minimum set cover problem. To yield acceptable running times of the solver, the Internet and word networks are reduced in size by extracting their high-degree cores of about 4,500 nodes. The Hungarian road data are processed slightly differently. First the cities in Hungary are mapped to their geographic coordinates using the database in http://www.kemitenpet.hu/letoltes/tables.helyseg_hu.xls . Then these coordinates are used in the GLPK to find the NNG equilibrium. Each edge in this equilibrium network is then checked for existence in the real road network. To check that, the GoogleMaps API https://pypi.python.org/pypi/googlemaps/ is used to find the shortest path between the two cities connected by the edge. The edge is defined to also exist in the real road network if this shortest path does not go via any other city. How to cite this article : Gulyás, A. et al. Navigable networks as nash equilibria of navigation games. Nat. Commun. 6:7651 doi: 10.1038/ncomms8651 (2015).